Reinforcement of hydrogels using three-dimensionally printed microfibres Despite intensive research, hydrogels currently available for tissue repair in the musculoskeletal system are unable to meet the mechanical, as well as the biological, requirements for successful outcomes. Here we reinforce soft hydrogels with highly organized, high-porosity microfibre networks that are 3D-printed with a technique termed as melt electrospinning writing. We show that the stiffness of the gel/scaffold composites increases synergistically (up to 54-fold), compared with hydrogels or microfibre scaffolds alone. Modelling affirms that reinforcement with defined microscale structures is applicable to numerous hydrogels. The stiffness and elasticity of the composites approach that of articular cartilage tissue. Human chondrocytes embedded in the composites are viable, retain their round morphology and are responsive to an in vitro physiological loading regime in terms of gene expression and matrix production. The current approach of reinforcing hydrogels with 3D-printed microfibres offers a fundament for producing tissue constructs with biological and mechanical compatibility. Hydrogels are an important class of biomaterials with many applications, including as cell carriers for the engineering of tissues [1] , [2] . In this respect, hydrogels are designed to provide the cells with a fully hydrated three-dimensional (3D) environment comparable to the extracellular matrix of native tissues [3] , [4] . When embedded within hydrogels, cells need to form a tissue-specific matrix that is capable of repairing or regenerating the damaged tissue. However, hydrogels often have inadequate mechanical properties, which are either unfavourable to embedded cells or make them too weak for application in the musculoskeletal system [5] , [6] , [7] . The performance of hydrogel implants is expected to be superior when they closely match the mechanical properties of their target tissue [8] , [9] . This is based on the principle that cells in native tissues are responsive to different types of mechanical stresses, such as compression, tension and shear [10] , [11] , [12] . These properties, for example stiffness, can be improved by increasing the hydrogel polymer concentration or crosslink density [2] , [3] , [13] or by the formation of tissue-specific extracellular matrix before implantation of the graft [2] , [14] , [15] . However, this generally compromises the biological performance of the hydrogel [2] , [3] or requires a long and costly period of pre-culture. Tissue engineers have, therefore, been inspired by the architecture of native tissues, which derive their unique mechanical properties from a fibrous protein framework that supports the aqueous component, forming a complex composite [16] . For example, hydrogels have been reinforced with nanofibres [17] , [18] , [19] , microfibres [20] and woven [8] , [21] , [22] or non-woven [23] scaffolds. The mechanical properties of hydrogels in such composites are less demanding; therefore, they can be processed with a low crosslink density, which is beneficial for cell migration and the formation of neo-tissue [2] , [3] . Recent composite systems include non-woven scaffolds manufactured via solution-electrospinning techniques [9] , [24] , [25] , [26] , [27] and scaffolds fabricated via 3D-printing [28] , [29] , [30] , [31] , [32] , [33] . Owing to the small fibre diameters that can be obtained, electrospun meshes have the potential to mimic native tissue extracellular matrix structures, including its mechanical properties. However, a disadvantage of traditional solution electrospinning techniques is the limited control over network architecture. Recently, melt electrospinning has been used in a direct writing mode, and may overcome this limitation, with the layer-by-layer assembly of the low-diameter fibres, permitting tight control over the network architecture [34] , [35] . This study aims to mechanically reinforce gelatin methacrylamide (GelMA) hydrogels with organized, high-porosity poly(ɛ-caprolactone) (PCL) fibre scaffolds. GelMA is a hydrogel platform with recent use that allows for matrix deposition by embedded cells, for example, vascular networks or cartilage matrix [14] , [36] , [37] . Reinforcing scaffolds with different porosities are fabricated from medical-grade PCL by melt-electrospinning in a direct writing mode [34] . Fibrous hydrogel composites are then fabricated by infusing and crosslinking GelMA within the PCL scaffolds. The stiffness and recovery under cyclic compression of these composites are analysed depending on PCL scaffold porosity and the degree of crosslinking of the GelMA. A mathematical model is developed using the scaffold parameters, and subsequently used to simulate and predict the degree of hydrogel reinforcement. Finally, human primary chondrocytes are encapsulated in the composite constructs and their viability, morphology and chondrogenic differentiation were investigated in an in vitro culture assay under physiological compressive loading. We demonstrate that hydrogels are reinforced in a synergistic manner with high-porosity microfibre scaffolds. The stiffness of the composites approaches that of articular cartilage, while maintaining a relevant elasticity. Chondrocytes embedded in the composite constructs respond positively to a repetitive mechanical loading regime in a bioreactor culture, in terms of cartilage gene expression and matrix formation. These hydrogel/microfibre composites thus offer a mechanically and biologically favourable environment for the engineering of tissues. Fabrication of PCL microfibre scaffolds PCL scaffolds of 1 mm height were 3D-printed with a reproducible quality using melt-electrospinning writing ( Fig. 1a and Supplementary Movie 1 ). Scaffolds were fabricated with fibre spacings between 0.2 mm ( Fig. 1b ) and 1.0 mm ( Fig. 1c ). The fibres were well aligned and fused at the 0°- to 90°-oriented junctions ( Fig. 1d ). The fidelity of fibre deposition decreased for constructs higher than 1 mm, probably because of the electric isolating effect of the scaffold that had already been deposited on the collector plate. Therefore, two scaffolds were stacked in the current study to obtain 2-mm-high constructs. The scaffold porosity could be controlled within the range of 93–98% by varying the set fibre spacing between 0.2 and 1.0 mm ( Fig. 1e ). Flow rates of 18, 72 and 180 μl h −1 corresponded to fibre diameters of 19.4±1.7, 48.5±8.2 and 88.5±7.6 μm, respectively. Larger diameter scaffolds of the same polymer were 3D-printed with traditional melt extrusion-based methods as a control for the mechanical analyses. These scaffolds had a fibre diameter of 219.7±14.2 and a porosity ranging from 89 to 72%, depending on the set fibre spacing. 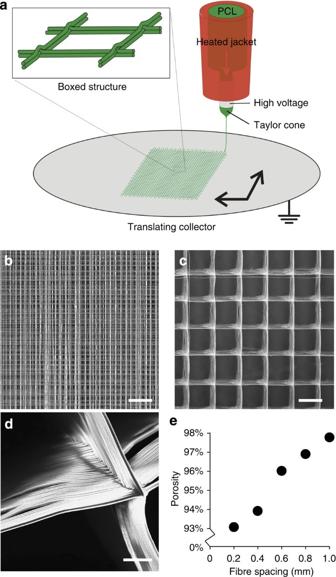Figure 1: Fabrication of microfibre scaffolds. 3D scaffolds were fabricated from PCL by 3D printing, that is, melt-electrospinning in a direct writing mode. (a) Thin PCL fibres were stacked in a 0–90° orientation through combined extrusion and an electrostatic field between the dispensing needle and the translating collector plate. Several fibre spacings were applied ranging from (b) 0.2 and (c) 1.0 mm as visualized with stereomicroscopy (scale bar, 1 mm). (d) Detailed image of the fibres that fused at the cross-sections (fibre spacing 1.0 mm, scale bar, 200 μm). (e) The porosity of the scaffolds varied between 93 and 98% depending on the set fibre spacing. Figure 1: Fabrication of microfibre scaffolds. 3D scaffolds were fabricated from PCL by 3D printing, that is, melt-electrospinning in a direct writing mode. ( a ) Thin PCL fibres were stacked in a 0–90° orientation through combined extrusion and an electrostatic field between the dispensing needle and the translating collector plate. Several fibre spacings were applied ranging from ( b ) 0.2 and ( c ) 1.0 mm as visualized with stereomicroscopy (scale bar, 1 mm). ( d ) Detailed image of the fibres that fused at the cross-sections (fibre spacing 1.0 mm, scale bar, 200 μm). ( e ) The porosity of the scaffolds varied between 93 and 98% depending on the set fibre spacing. Full size image Stiffness of reinforced GelMA and alginate hydrogels A synergistic effect was observed on construct stiffness (strain rate 25% min −1 ) when GelMA and alginate hydrogels were reinforced with the microfibre PCL scaffolds ( Fig. 2 ). The stiffness of PCL scaffolds alone increased from 1.1±0.3 kPa for 98% porosity to 15.2±2.2 kPa for the 93% porosity scaffold ( Fig. 2a ). The stiffness of the scaffolds was comparable to that of hydrogels: 7.1±0.5 and 7.5±1.0 kPa for GelMA crosslinked with either 12.5 or 25 m M ammonium persulfate/tetramethylethylenediamide (APS/TEMED) and 15.8±2.0 kPa for alginate ( Fig. 2b ). When the compressive strength of the 93% porous PCL/hydrogel composite was investigated, the construct stiffness was increased 30-fold, up to 214±24 kPa for GelMA with 12.5 m M APS/TEMED, and 54-fold, up to 405±68 kPa, when the GelMA was crosslinked with 25 m M APS/TEMED ( Fig. 2c,d ). Alginate hydrogels also showed synergistic reinforcement (15-fold up to 240.7±37.8 kPa) that was comparable to GelMA gels ( Fig. 2e ). The reinforcing effect in the composites was dependent on the porosity of the PCL scaffold, which ranged from 93 to 98%. Interestingly, increasing the fibre roughness and surface area by etching of the PCL scaffold did not increase the degree of reinforcement ( Supplementary Fig. 1 ). In fact, prolonged etching times resulted in mass loss of PCL, and hence decreased the construct stiffness. Therefore, we concluded that the strength increase seen in the composites was not due to hydrogel/fibre bonding. 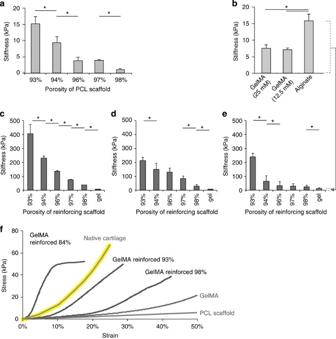Figure 2: Reinforcing effect of high-porosity 3D-printed PCL scaffolds incorporated into hydrogels. (a) Compressive moduli of PCL scaffolds were in the same range as those of (b) hydrogels alone. GelMA reinforced with PCL scaffolds and crosslinked with either (c) 25 mMor (d) 12.5 mMAPS/TEMED were one order of magnitude stiffer than the scaffolds or gel alone; (e) a comparable degree of reinforcement for reinforced alginate gels (*P<0.05, one-way ANOVA with Bonferroni correction). (f) Stress–strain curves of GelMA, the PCL scaffold and reinforced GelMA, approaching the curve of native cartilage (yellow). Scaffolds fabricated from thick fibres (that is, 84%) were stiffer than native cartilage, but often disintegrated at a strain of∼10% (all groupsn=5, mean±s.d.; cartilagen=8). Here GelMA was crosslinked with 12.5 mMAPS/TEMED and the strain rate applied was 25% min−1. Figure 2: Reinforcing effect of high-porosity 3D-printed PCL scaffolds incorporated into hydrogels. ( a ) Compressive moduli of PCL scaffolds were in the same range as those of ( b ) hydrogels alone. GelMA reinforced with PCL scaffolds and crosslinked with either ( c ) 25 m M or ( d ) 12.5 m M APS/TEMED were one order of magnitude stiffer than the scaffolds or gel alone; ( e ) a comparable degree of reinforcement for reinforced alginate gels (* P <0.05, one-way ANOVA with Bonferroni correction). ( f ) Stress–strain curves of GelMA, the PCL scaffold and reinforced GelMA, approaching the curve of native cartilage (yellow). Scaffolds fabricated from thick fibres (that is, 84%) were stiffer than native cartilage, but often disintegrated at a strain of ∼ 10% (all groups n =5, mean±s.d. ; cartilage n =8). Here GelMA was crosslinked with 12.5 m M APS/TEMED and the strain rate applied was 25% min −1 . Full size image Comparison of reinforced gels with articular cartilage The average stress–strain curve of native cartilage samples (strain rate 25% min −1 ; n =8) that were harvested from the patellofemoral groove of an equine knee joint was plotted in Fig. 2f together with the average ( n =5) stress–strain curves for GelMA, high-porosity PCL scaffolds and GelMA reinforced with 98%, 93% and 84% porosity PCL scaffolds, respectively. Clearly, GelMA gels were much softer than the cartilage. However, the stiffness and deformation profile (shape of the stress–strain curve) of GelMA could be tailored to that of native cartilage by reinforcement with high-porosity PCL scaffolds. While thick-fibre scaffolds (porosity 72–88%), as fabricated with traditional 3D-printing methods, were stiffer than native cartilage, they broke at ∼ 10% strain when large fibre spacings were applied (>1.25 mm). This sudden loss of integrity was not observed for native cartilage or gels reinforced with high-porosity scaffolds ( Fig. 2f ). Time-dependent stress response of reinforced gels and cartilage The stress response to isostrain showed that GelMA reinforced with a 93% porosity scaffold has a higher modulus on initial loading than cartilage ( Fig. 3 ). However, relaxation is faster, and to a lower equilibrium modulus, than cartilage. The modulus of GelMA was much lower during the isostrain at any time. 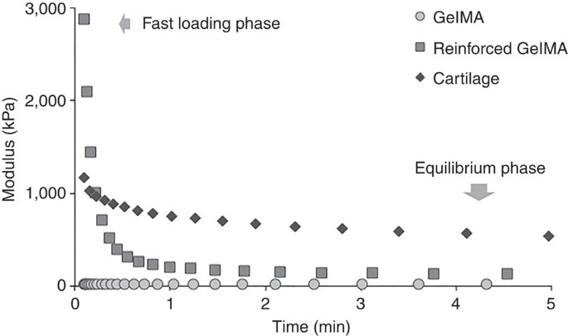Figure 3: The time-dependent stress response of (reinforced) GelMA gel and articular cartilage at 9% isostrain. Reinforced GelMA displays a high modulus compared with cartilage on direct loading. The modulus of reinforced gels in the equilibrium phase, however, is closer to gel than to cartilage. These plots are representative for the series of isostrains that were consecutively performed for 15 min. Analysis of the stress curves at isostrain indicated that the reinforced GelMA constructs could not be adequately described within an isotropic poroelastic framework, but that a bi-exponential function: Figure 3: The time-dependent stress response of (reinforced) GelMA gel and articular cartilage at 9% isostrain. Reinforced GelMA displays a high modulus compared with cartilage on direct loading. The modulus of reinforced gels in the equilibrium phase, however, is closer to gel than to cartilage. These plots are representative for the series of isostrains that were consecutively performed for 15 min. Full size image provided an accurate, phenomenological characterization of the time-dependent response of the construct, where S is the stress, t is time and the constants S i and K i have units of stress and time, respectively. A nonlinear least squares fitting algorithm was used to obtain the best fitting parameters for S i and K i from the 9% isostrain curves as detailed in Supplementary Fig. 2 and Supplementary Note 1 . We report E i = S i /strain as elastic moduli, so that E 0 is the equilibrium modulus and E 1 and E 2 are ‘transient’ moduli that characterize the time-dependent response of the material so that the ‘peak’ equilibrium modulus is obtained by summing the E i ( Table 1 ). Table 1 Fit of a bi-exponential function to the time-dependent stress response. Full size table Modelling the fibre reinforcement of hydrogels The mechanism we propose to explain the synergistic reinforcement is illustrated in Fig. 4a . Hydrogels can be reasonably described as incompressible [38] ; therefore, the volume of the hydrogel is conserved and vertical compression must be accompanied by horizontal expansion. As a composite construct is loaded, each ‘semi-confined cell’ of hydrogel (right column in Fig. 4a ) expands horizontally and places the surrounding fibres under tension. We hypothesize that the fibres’ resistance to elongation under compression loading results in a pre-stress of the scaffold fibres. This resistance leads to the observed increase in stiffness, as the stiffness of bulk PCL is approximately four orders of magnitude higher than that of the gels. 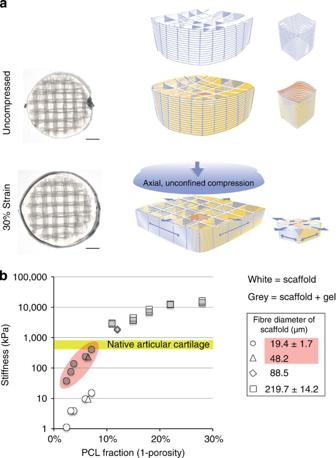Figure 4: The mechanism of hydrogel reinforcement with organized high-porosity scaffolds. (a) PCL microfibre scaffolds (blue in schematic) serve as a reinforcing component to GelMA hydrogel (yellow in schematic). When axial compression is applied to the reinforced hydrogels, the stiff thin scaffold fibres stretch on lateral displacement of the hydrogel. This mechanism provides the composites with a high stiffness and elasticity (scale bars, 1 mm). (b) Moduli of scaffolds and scaffold/gel composites as a function of porosity, showing the synergistic increase in stiffness was only observed for thin-fibre scaffolds with a high porosity (polymer fraction 2–7%=porosity 98–93% (highlighted in red)), fabricated with melt-electrospinning writing (MEW). Fused deposition modelling (FDM) scaffolds were fabricated from 10-fold thicker fibres, resulting in a higher stiffness; however, no synergistic reinforcement was observed (mean ofn=5). In order to confirm our hypothesis, we developed a mathematical model that enables us to make the following prediction for the construct stiffness, C : Figure 4: The mechanism of hydrogel reinforcement with organized high-porosity scaffolds. ( a ) PCL microfibre scaffolds (blue in schematic) serve as a reinforcing component to GelMA hydrogel (yellow in schematic). When axial compression is applied to the reinforced hydrogels, the stiff thin scaffold fibres stretch on lateral displacement of the hydrogel. This mechanism provides the composites with a high stiffness and elasticity (scale bars, 1 mm). ( b ) Moduli of scaffolds and scaffold/gel composites as a function of porosity, showing the synergistic increase in stiffness was only observed for thin-fibre scaffolds with a high porosity (polymer fraction 2–7%=porosity 98–93% (highlighted in red)), fabricated with melt-electrospinning writing (MEW). Fused deposition modelling (FDM) scaffolds were fabricated from 10-fold thicker fibres, resulting in a higher stiffness; however, no synergistic reinforcement was observed (mean of n =5). Full size image where N f denotes the number of fibres in the construct, E the Young's modulus of the reinforcing polymer, ρ the fibre radius, R the construct radius and λ the axial strain (expressed as a fraction of the initial height). A derivation and more detailed explanation of the model are provided in the Supplementary Table 1 and Supplementary Note 2 . Video analysis of the compression cycle of reinforced gels The model was further validated by lateral video imaging of the compression cycle of the GelMA/PCL composites, which revealed elongation (stretching) of PCL microfibres and a concave profile at the sides of the construct because of lateral displacement of water from GelMA ( Supplementary Movie 2 , 97% porosity scaffold). The microfibres stretched 9±1% on 30% axial strain. In addition, from a top view it was observed that the PCL scaffold area expanded 17% and the aqueous component expanded 23% (including exudation of water; Fig. 4a ). Microfibre compared with thick-fibre composites The reinforcing effect was only observed in high-porosity scaffolds fabricated from thin fibres (diameter <48.2 μm), as indicated in Fig. 4b . The 3D-printing of thicker fibres (diameter >88.5 μm) resulted in a significantly lower scaffold porosity, ranging from 88 to 72% (PCL fraction of 12% to 28%, respectively), depending on the fibre thickness and spacing between the fibres. The stiffness of the thick-fibre scaffolds ranged from 1.8±0.2 MPa for 88% porosity to 16.1±1.7 MPa for 72% porosity. These scaffolds had stiffnesses similar to those of their composite counterparts with crosslinked GelMA. The compression cycle of GelMA reinforced with an 82% porosity scaffold is shown in Supplementary Movie 3 . Exudation of fluid was observed; while the relatively thick scaffold fibres were compressed, they did not elongate. Recovery of GelMA constructs after compression The recovery of (reinforced) GelMA constructs after repetitive axial compression was measured. 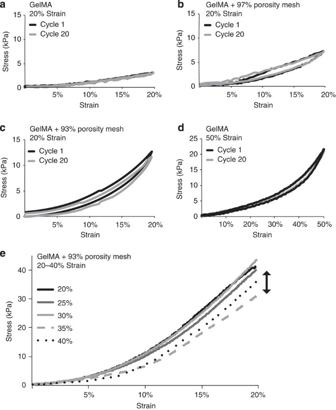Figure 5: Cyclic compression testing of GelMA and reinforced GelMA constructs. The stress–strain curves of the first and last of 20 cycles of 20% compression are shown for (a) GelMA alone, (b) GelMA reinforced with a 97% porosity PCL scaffold and (c) GelMA reinforced with a 93% porosity PCL scaffold. For all groups no decay in stress was observed. (d) GelMA constructs also recovered after 20 cycles of 50% axial compression; however, (e) GelMA reinforced with a 93% porous PCL scaffold required substantially less force to be compressed to 20% strain, after being compressed to over 30% strain (arrow; mean ofn=3). Figure 5a–c shows that GelMA, as well as reinforced GelMA constructs, are fully elastic after 20 cycles of 20% strain. The stress–strain curves of the initial and final loading cycle are shown. GelMA also fully recovered after repetitive 50% axial strain ( Fig. 5d ). However, GelMA reinforced with 93% porosity PCL microfibre scaffolds showed significantly decreased resistance when axially deformed by over 35% ( Fig. 5e ). Figure 5: Cyclic compression testing of GelMA and reinforced GelMA constructs. The stress–strain curves of the first and last of 20 cycles of 20% compression are shown for ( a ) GelMA alone, ( b ) GelMA reinforced with a 97% porosity PCL scaffold and ( c ) GelMA reinforced with a 93% porosity PCL scaffold. For all groups no decay in stress was observed. ( d ) GelMA constructs also recovered after 20 cycles of 50% axial compression; however, ( e ) GelMA reinforced with a 93% porous PCL scaffold required substantially less force to be compressed to 20% strain, after being compressed to over 30% strain (arrow; mean of n =3). Full size image Chondrogenic differentiation of embedded human chondrocytes Haematoxylin and eosin-stained sections revealed that chondrocytes retained their spherical morphology within the fibre-reinforced hydrogels after 7 days ( Fig. 6c ). Chondrocytes were also homogenously distributed throughout the construct as shown by the 4′,6-diamidino-2-phenylindole (DAPI)-stained cell nuclei ( Fig. 6d ). Chondrocytes maintained high cell viability on days 1 and 7 when crosslinked with 12.5 m M APS/TEMED ( Fig. 6e ). Following 14 days of culture, hydrogels (GelMA with 0.5% hyaluronic acid (Lifecore, USA; GelMA-HA) for improved chondrogenic differentiation [14] and GelMA-HA with 93% porous PCL mesh) were subjected to physiological loading cycles for another 14 days. The stress response to the 1 Hz dynamic loading regime is presented in Supplementary Fig. 3 . Analysis of the quantitative reverse transcriptase–PCR (qRT–PCR) data indicated that for chondrocytes within the fibre-reinforced hydrogels, ACAN (gene expression for glycosaminoglycan (GAG) synthesis) and COL1A1 (gene expression for collagen type I) mRNA levels were significantly upregulated in the compressed (‘C’) groups compared with the control, non-compressed groups (‘NC’; Fig. 6f–i ; P <0.05). Further, chondrocytes in the reinforced gels were more responsive to loading regime than cells in GelMA alone. Stiffness values were ∼ 400 kPa in cell-laden fibre-reinforced hydrogels ( Fig. 6j ). There was no significant effect of reinforcement or compression on construct stiffness and glycosaminoglycan (GAG) content ( Fig. 6k ). The chondrocytes within the gels exhibited pericellular collagen type I and II deposition in all groups, with no discernible differences between the groups ( Supplementary Fig. 4 ). 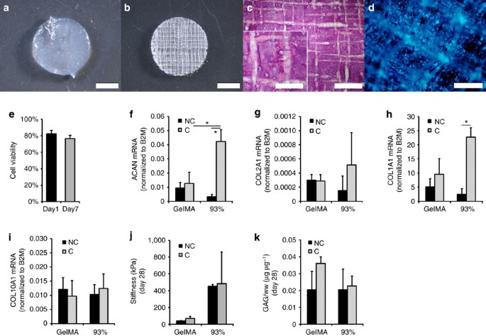Figure 6: Differentiation of chondrocytes embedded in reinforced GelMA-HA hydrogels. (a) Stereomicroscopy image of a GelMA-HA gel and (b) of a GelMA-HA gel reinforced with a PCL scaffold (93% porosity) on day 1 (scale bars, 2 mm). (c) Haematoxylin/eosin staining after 7 days of culture shows that chondrocytes remained within the GelMA component and retained a round morphology (scale bar, 500 μm, inlay, 200 μm). (d) DAPI staining confirms a homogenous distribution of the cells throughout the construct (scale bar, 200 μm). (e) Chondrocytes remained viable over 7 days of culture in the gels. Gene expression analysis for (f) ACAN, (g) COL2A1, (h) COL1A1 and (i) COL10A1 on day 14 for compressed (C) and non-compressed (NC) groups (n=4, mean±s.d.; *P<0.05, two-way ANOVA). All gene expression levels were normalized to the housekeeping gene β2 microglobulin (B2M). (j) Stiffness of the constructs following long-term culture (n=4). (k) GAG/ww values on day 28 (n=5). Figure 6: Differentiation of chondrocytes embedded in reinforced GelMA-HA hydrogels. ( a ) Stereomicroscopy image of a GelMA-HA gel and ( b ) of a GelMA-HA gel reinforced with a PCL scaffold (93% porosity) on day 1 (scale bars, 2 mm). ( c ) Haematoxylin/eosin staining after 7 days of culture shows that chondrocytes remained within the GelMA component and retained a round morphology (scale bar, 500 μm, inlay, 200 μm). ( d ) DAPI staining confirms a homogenous distribution of the cells throughout the construct (scale bar, 200 μm). ( e ) Chondrocytes remained viable over 7 days of culture in the gels. Gene expression analysis for ( f ) ACAN, ( g ) COL2A1, ( h ) COL1A1 and ( i ) COL10A1 on day 14 for compressed (C) and non-compressed (NC) groups ( n =4, mean±s.d. ; * P <0.05, two-way ANOVA). All gene expression levels were normalized to the housekeeping gene β2 microglobulin (B2M). ( j ) Stiffness of the constructs following long-term culture ( n =4). ( k ) GAG/ww values on day 28 ( n =5). Full size image In this study, high-strength composite constructs were fabricated by combining 3D-printed high-porosity scaffolds with a hydrogel. These composite hydrogels can be customized to yield a wide range of mechanical properties and, from a biological point of view, have the capacity to support cell proliferation and extracellular matrix production. The PCL scaffolds were built by micrometre-scale fibres that were organized and interconnected through the melt-electrospinning writing process. With this unique and new 3D-printing technique, pre-set network architectures can be realized in a direct writing mode [34] . This technique allows fibres to be printed well below the limits of classical melt-extrusion-based 3D-printing technologies such as fused deposition modelling [39] , with filament diameters as small as 5 μm, instead of 100 μm or larger [35] . Hydrogels have previously been reinforced with solution-electrospun nonwovens [9] , [24] , [25] , [27] . However, most traditional solution-electrospun meshes have disadvantages from both a mechanical and biological point of view, for example, fibres are not fused and hence slide under loading meshes are usually not thicker than 100 μ and have a pore size of less than 5 μm and are, therefore, too dense for cell infiltration [25] , [27] , [40] . To overcome these issues related to traditional solution electrospinning, fibres have been collected in an earthed ethanol bath, yielding nonwovens with high porosities [9] , [24] . Hydrogel stiffness was increased fourfold when reinforced with these randomly organized nonwovens, irrespective of the porosity [24] , [25] . Silk microfibres [20] or carbon nanotubes [17] also formed porous reinforcing structures for hydrogels, permitting cellular infiltration and differentiation. However, the stiffness of the gels increased only one- to threefold, as the fibres were not fused. In contrast, in our current composite model consisting of a relatively soft hydrogel (7.1–15.8 kPa) and a highly porous and soft PCL scaffold (1.1–15.2 kPa), the maximum stiffness obtained was a factor of 50 larger (405 kPa) than that of the hydrogels alone, on a strain rate of 25% min −1 . The stiffness of cartilage and (reinforced) hydrogels is strongly strain-rate-dependent [41] , [42] . We found that the reinforced hydrogels were one order of magnitude stiffer than cartilage on initial fast loading at 9% strain. However, the modulus of reinforced hydrogels displayed a steep decrease to an equilibrium value roughly one-third the equilibrium modulus of cartilage, yet still one order of magnitude larger than the equilibrium modulus of hydrogel alone. The effect of reinforcement can be explained by the highly organized fibre architecture of the scaffolds. The mathematical model we developed demonstrated that the hydrogel places the PCL fibres under tension on axial compression, and predicts a theoretical upper bound on the attainable stiffness. However, the theoretical stiffness of the reinforced hydrogels is one order of magnitude larger than that observed experimentally. This is reasonable since an idealized construct was considered, in which the fibres are initially taut at zero strain, the hydrogel is purely elastic and there is no slip between the fibres and the hydrogel. In fact, in our experimental set-up, we showed that very little water, or hydrogel, was compressed out of the constructs; therefore, the fibres did not completely lock the hydrogel. The stress relaxation on isostrain ( Fig. 3 ) reflects the exudation of the aqueous component (water or gel) from the reinforcing scaffold. For cartilage we observed a higher equilibrium modulus, which may be a combined effect of the osmotic pressure of fixed charges on proteoglycans and an organized extracellular matrix. Etching the high-porosity scaffolds did not result in a further increase in stiffness of the composites. This approach was on the basis of our previous finding that covalent attachment of the hydrogel component to a scaffold that was fabricated from modified, methacrylated PCL, resulted in increased construct strength [29] . It should be noted that etching results in an increase in van de Waals forces but does not establish covalent bonds between the hydrogel and the reinforcing scaffold. Infiltrating hydrogel into scaffolds that had been fabricated with traditional 3D melt-printing techniques with thick fibres (≥88 μm) [39] did not show a significant mechanical effect. Axial loading of these constructs requires compression of the PCL through a strong vertical column of fibre crossings, which is not easily deformed. Video imaging of the compression cycle confirmed that thick fibres were not stretched and water flowed out of these scaffolds without providing a synergistic effect. In contrast, the columns of fine fibre crossings are easily deformed under axial loading; however, they are supported by the hydrogel component in the composites. Supplementary Movie 2 shows some local distortion of the columns, but no large-scale buckling of the columns; therefore, the microfibres are put under tension. We further note that this axial loading reduces the horizontal pore size, improving gel confinement. To our knowledge, we are the first to show the synergistic effect of a well-designed scaffold/hydrogel system; the work shown in this paper could therefore lead to a paradigm shift in the field. Reinforced GelMA hydrogels possess stress–strain curves that closely resemble those of healthy articular cartilage. In addition, in absolute terms, the stiffness of the biodegradable composites was comparable to the stiffness of articular cartilage, which has been reported to range from 400 to 800 kPa (refs 43 , 44 , 45 ). On the other hand, the stiffness of scaffolds fabricated with traditional 3D-printing was one order of magnitude larger than that of the articular cartilage, which is consistent with previous reports [30] , [33] . The porosity of these scaffolds ranged between 72 and 89%, whereas the porosities reported in the literature range from 28.9 and 91.2% (refs 39 , 46 , 47 ). Nevertheless, when aiming to fabricate high-porosity scaffolds (>80%) from thick fibres, large fibre spacing (>1.5 mm) is required, which causes scaffold disintegration under strains of ∼ 10%. In addition, the thicker fibres occupy a relatively high volume that is inaccessible for tissue formation until the scaffold has degraded. Hydrogels reinforced with woven scaffolds, composed of either polyglycolic acid [8] or PCL [21] , [22] , have previously been reported to possess tensile, compressive and shear properties comparable to native cartilage. The porosity of these woven scaffolds was 70–74%, compared with 93–98% in the present study. The stiffness of the woven composites was reported up to 0.2 Mpa (at equilibrium stress), which was twice as stiff as the scaffold without the gel [22] . Both the woven and the melt-electrospun composites showed axial recovery after compression for 10% and 20%, respectively. The water that was compressed out of the scaffolds was likely reabsorbed during the relaxation phase, comparable to fluid dynamics in the articular cartilage [48] . Our reinforced hydrogels showed decreased resistance if compressed by 35% or more, which may be because of fractures or delamination in the PCL scaffold junctions. For translational purposes, it is important to realize that native cartilage is exposed to 15–45% axial deformation under long-term static compression [49] . Incorporation of organized fibrous PCL scaffolds within a well-characterized hydrogel system makes it possible to culture cells in a customizable, mechanically diversified environment. The hydrogel component of the composite constructs will degrade within months [14] , [29] , allowing the regeneration of new tissue, while the PCL component degrades within years [50] forming a temporary reinforcing network to the new tissue. Under physiological compressive loading of 20% strain and 1 Hz, our gene expression data suggest that chondrocyte expression of matrix mRNAs is significantly upregulated in composite hydrogels compared with non-reinforced, weak hydrogels. These results highlight the importance of developing cell-culture platforms and tissue-engineered constructs that better mimic the in vivo mechanoenvironment of natural articular cartilage. Still, the exact mechanisms of stress transfer to the cells in fibre-reinforced hydrogels remain to be investigated. In conclusion, the current work represents a significant step towards developing biomechanically functional tissue constructs. The stiffness of the constructs was significantly enhanced, achieving values similar to those of native articular cartilage, by combining hydrogels with 3D-printed, high-porosity melt-electrospun PCL scaffolds. This synergistic effect could be modulated by altering the porosity of the reinforcing scaffolds. The composite constructs have a strong elastic component and recover after physiological axial strains. Finally, human chondrocytes encapsulated in the GelMA/PCL composites were found to be more responsive to mechanical loading, which led to significant changes in gene expression in vitro . Fabrication of PCL microfibre scaffolds Several scaffolds were 3D-printed from medical-grade PCL (PURAC, Gorinchem, the Netherlands) with a custom-made melt-electrospinning device [34] . PCL was heated to 103 °C in a 2 ml polypropylene syringe and extruded at a rate of 18 μl h −1 using a syringe pump. In combination with an electrostatic field of 8–10 kV between the syringe needle tip (23G) and the collector plate (3 cm distance), a stable PCL jet was obtained. Defined scaffold architectures, with dimensions up to 120 × 120 × 1 mm, were realized through computer-aided movement of the aluminium collector plate at a speed of 1,400 mm min −1 , using the Mach3 motion control software (Artsoft, USA). A predefined 0–90° architecture was imposed, with a fibre spacing of 0.2, 0.4, 0.6, 0.8 or 1.0 mm. The melt-electrospinning writing was terminated when scaffolds reached a height of 1.0 mm, to ensure maximum quality of the architecture. To investigate the effect of the PCL flow rate on fibre diameter and scaffold porosity, we printed constructs at 4 × and 10 × flow rate, with a fibre spacing of 0.4 and 1.0 mm, respectively. Cylindrical samples were extracted from the scaffolds with a 5-mm diameter biopsy punch. Two scaffolds were stacked in order to achieve a height of 2 mm, which is comparable to the thickness of human cartilage in the knee joint [51] . The porosity and mechanical properties of the melt-electrospun scaffolds were compared with scaffolds fabricated with traditional 3D-printing technologies. To this end, scaffolds were 3D-printed from PCL with a BioScaffolder system (SYS+ENG, Salzgitter-Bad, Germany) as described previously [46] . Briefly, PCL was heated till 70 °C and extruded with an Auger screw through a 27-gauge needle. Scaffolds measuring 40 × 40 × 2 mm were fabricated with a fibre spacing of 0.75, 1.0, 1.25, 1.5 and 1.75 mm. The quality of the scaffolds was imaged both with stereomicroscopy and Scanning Electron Microscopy (SEM, Hitachi TM3000, Japan and Quanta 200, FEI, Milton, Australia). The fibre diameter was measured with the ImageJ software (National Institutes of Health, USA). The porosity of the PCL scaffolds was determined gravimetrically. Etching of PCL microfibre scaffolds PCL scaffolds were etched in order to increase its hydrophilicity and surface area, which could potentially contribute to the stiffness of reinforced GelMA constructs. Cylindrical PCL scaffolds with a porosity of 94% were treated with 70% ethanol and subsequently etched with 5 M sodium hydroxide for 0, 1, 2, 4, 8 and 16 h. After etching, the scaffolds were washed in deionized H 2 O until the pH reached 7.4, and then air-dried. The effect of etching was evaluated by measuring the fibre diameter (ImageJ) from SEM images, and by assessing the weight from 2 × 5 mm diameter scaffolds (expressed in relative weight loss). Since mild etching will increase hydrophilicity and may facilitate perfusion of GelMA through the PCL scaffold, 2 h of etching was performed for all other experiments presented. Preparation of GelMA and alginate gels GelMA was synthesized by reaction of type A gelatin (Sigma-Aldrich, St Louis, MO, USA) with methacrylic anhydride at 50 °C for 1 h as previously described [14] . GelMA was dissolved in PBS at 60 °C at a concentration of 10% (w/v) containing 12.5 or 25 m M APS. TEMED (12.5 or 25 m M ) was added followed by 5 s vortexing in order to initiate crosslinking of the GelMA. Sodium alginate (IMCD, Amersfoort, the Netherlands) was dissolved in PBS at 3% (w/v), and used as a control gel to GelMA for the mechanical analyses. Preparation of reinforced hydrogel constructs The scaffolds were placed in an injection mold that was custom-made from polymethylmethacrylate in order to fit 10 cylinders with a diameter of 5 mm and a height of 2 mm. All cylindrical voids in the mold were interconnected so that gel could be serially perfused. The mold was sealed with a sheet of polyethylene that was fixed between two glass histology slides. Directly after mixing in the TEMED, the GelMA solution as described above was injected in the mold untill all PCL scaffolds were fully infused. Crosslinking of the GelMA was allowed in this mold at 37 °C for 1 h. Cell-free samples were then stored in PBS at 37 °C. Chondrocyte-laden samples were kept in a chondrocyte expansion medium. In order to evaluate the effect of etching time of the scaffolds on construct stiffness, GelMA was reinforced with scaffolds etched for 0–16 h (all n =5) and crosslinked with 25 m M APS/TEMED. In addition, 93–98% porosity PCL scaffolds (all n =5) were infused with alginate in the mold. The alginate composite constructs were then crosslinked by immersion in a 102-mmol calciumchloride solution for 30 min. Harvest of equine cartilage Full-thickness cartilage was harvested from the knee joint from one equine donor (10 years old) with macroscopically healthy cartilage. This was performed after consent of the horse owner and according to the ethical guidelines of the Utrecht University. Equine cartilage was used because of the availability and its similarities to human cartilage [51] . Cylindrical samples with a diameter of 5 mm and a height of 2 mm ( n =8) were taken with a biopsy punch from the medial patellofemoral groove and stored in PBS for up to 3 h. Mechanical analyses The stiffness (or compressive modulus) of GelMA and alginate hydrogels, PCL scaffolds, the composite constructs and articular cartilage (all n =5) was measured by single uniaxial unconfined compression in air at room temperature, after 1–3 days of submersion in PBS from their preparation. We confirmed that for single-cycle compression testing, the absence of a PBS immersion bath does not influence the stress responses of hydrogel samples. The effect of crosslinking with 12.5 or 25 m M APS/TEMED was tested. The stress–strain curves of (reinforced) GelMA that was crosslinked with 12.5 m M APS/TEMED were compared with cartilage samples. Over a period of 2 min, a force ramp (axial strain rate ca. 25% min −1 ) was applied to the samples employing a microtester (Instron, Melbourne, Australia) or a Dynamic Mechanical Analyser (DMA 2980, TA Instruments, New Castle, DE, USA). The stiffness was calculated from the linear derivative of the stress–strain curve at 12–15% strain. In the low-porosity scaffolds that were fabricated with traditional 3D-printing, the 6–9% strain region was taken, as these constructs often disintegrated when strained beyond 10%. The compression cycle of GelMA reinforced with 97 and 82% porosity scaffolds was captured from the side (hand-held digital microscope 1.3 MP, Meade instruments, Europe GmbH & Co, Rhede, Germany) in order to analyse the lateral expansion of both components of the composite construct. In addition, images from the top of these constructs were taken with a stereomicroscope, when uncompressed and at 30% strain between two glass slides. In order to test the time-dependent stress response, GelMA, GelMA reinforced with 93% porosity scaffolds and articular cartilage samples were subjected to a series of isostrain steps [52] . Samples were 2% pre-strained for 5 min, followed by strains of 6, 9 and 13% that were consecutively applied for 15 min each. The experiments were performed in PBS and the stress response of all samples was recorded. The modulus on fast initial loading and the equilibrium modulus were extracted, and the stress decay rate was estimated by fitting to a bi-exponential function. The resistance to axial deformation of GelMA and GelMA reinforced with PCL constructs (porosity 93 and 97%) was measured after a cyclic (20 × ) axial strain of 20% (Allround-line Z020, Zwick Roell, Germany). In addition, the resistance after 20 cycles of axial deformation of 50% was measured for GelMA constructs. The recovery measurements were performed in PBS and constructs were allowed to recover for 1 min after every cycle. GelMA constructs reinforced with a 93% porous scaffold underwent compression with incremental maximum strains of 20–40% (with 5% increments) in order to analyse the maximal strain that could be exerted before irreversible damage would occur. Modelling the fibre reinforcement of hydrogels A mathematical model was constructed to investigate further the mechanisms by which the 3D-printed scaffolds reinforce the hydrogels. There is an extensive literature on the modelling of fibre-reinforced biological materials, with recent cartilage-focussed examples [41] , [42] . Fibre-reinforced materials are often modelled by assuming that it is reasonable to define a continuously varying fibre density and orientation and then making the material properties a function of these. In this instance, given that we know the arrangement and approximate number of fibres in each plane of the material, we take the more direct approach of considering how each fibre stretches as the scaffold deforms. Our model takes into account the number of fibres in the scaffold and the fibre diameter, the Young’s modulus of PCL and the construct dimensions. In the model, the composite construct was viewed as an elastic solid, in which the PCL fibres are placed under tension by the hydrogel on axial compression. Harvest of human chondrocytes Macroscopically healthy cartilage was harvested either from a discarded talus bone that was resected from a 7-year-old patient undergoing an orthopaedic intervention, or from the femoral condyles of knee replacement surgery patients (age: 71.0±4.1; n =6) with consent. This was in concordance with the institutional code of conduct regarding the use of discarded tissues in the University Medical Center Utrecht, and ethics approval was also obtained from Queensland University of Technology and Prince Charles hospital before sample collection. Cartilage was cut into small slices and washed with PBS supplemented with penicillin and streptomycin. The cartilage was digested overnight in 0.15% type II collagenase at 37 °C. The resulting cell suspension was filtered (100 μm cell strainer) and washed three times with PBS. Then, cells were resuspended in chondrocyte expansion medium (DMEM supplemented with 10% fetal bovine serum (FBS), 100 units ml −1 penicillin and 100 μg ml −1 streptomycin, and 10 ng ml −1 FGF-2) and expanded for 10 days in monolayer cultures (seeding density 5,000 cells cm −2 ). For the short-term study (7 day), chondrocytes from the talus bone were used at passage 2, and for the long-term study (28 day) chondrocytes obtained from the femoral condyles of the different donors were pooled and used at passage 1. Cell viability Chondrocytes were mixed in the GelMA/APS solution at a concentration of 10 million ml −1 . Crosslinking was performed with different proportions of APS/TEMED (12.5/12.5 and 25/25 m M ) in order to evaluate cytotoxicity of the redox crosslinking process. The viability of the chondrocytes was measured for 4 h (day 1) and 7 days after embedding and crosslinking of the GelMA constructs. To visualize cell viability, a LIVE/DEAD Viability Assay (Molecular Probes MP03224, Eugene, USA) was performed according to the manufacturer’s instructions. The samples were examined using a light microscope with the excitation/emission filter set at 488/530 nm to observe living (green) cells and at 530/580 nm to detect dead (red) cells. Photographs were taken with an Olympus DP70 camera. The ratio dead/alive was measured by assessing multiple parts of the sample. Cell morphology The morphology and location of chondrocytes in the reinforced GelMA constructs was assessed 7 days after encapsulation. Reinforced GelMA constructs with chondrocytes ( n =3, 93% porosity) were dehydrated through a graded ethanol series, cleared in xylene and embedded in paraffin. The samples were sectioned into 10-μm slices and stained with haematoxylin and eosine for the detection of GelMA, the PCL scaffold and the cells. In addition, the location of chondrocytes and their relation to the PCL fibres were assessed on days 1 and 7 with fluorescent staining withDAPI. To this end, constructs from GelMA only and reinforced with a PCL scaffold (93% porosity) were crosslinked with 12.5 m M APS/TEMED ( n =3). The GelMA was subsequently permeabilized with 1% Triton/PBS for 15 min and incubated with DAPI (0.1 μg ml −1 in PBS) for 5 min, followed by three washing steps with PBS. Fluorescence microscopy images were taken (with excitation/emission filter 330–385 nm) to detect the cell nuclei (blue). Mechanical stimulation For the chondrocyte redifferentiation experiment, 0.5% hyaluronic acid was added to 10% GelMA to promote redifferentiation of embedded chondrocytes [14] , [36] . Chondrocyte-laden GelMA-HA gels and GelMA-HA-PCL composite gels (PCL scaffold porosity: 93%) were able to swell freely under static conditions during the first 14 days. Following this pre-culture period, the constructs were cultured for another 14 days using a pre-established loading protocol (3 h per day, 20% strain, 1 Hz sinusoidal loading) in a commercial bioreactor (Cartigen C10-12c, Tissue Growth Technologies, Minnetonka, MN, USA). Constructs were cultured in high-glucose DMEM supplemented with 10 ng ml −1 transforming growth factor-β3, 1% insulin-transferrin-sodium (ITS), 1.25 mg ml −1 bovine serum albumin, 1 × 10 −7 M dexamethasone and other additives (GlutaMAX-1, 110 mg l −1 sodium pyruvate, 10 m M HEPES, 0.1 m M nonessential amino acides, 50 U ml −1 penicillin, 50 μg ml −1 streptomycin, 0.5 μg ml −1 fungizone and 0.1 m M L-ascorbic acid). Constructs were cultured for a total of 28 days. qRT–PCR Gene expression analysis was performed on the GelMA-HA hydrogels and the GelMA-HA hydrogels reinforced with 93% porosity PCL scaffold following 28 days of culture. RNA from the C and NC constructs was purified using the TRIzol reagent ( n =4). cDNA synthesis was carried out using the SuperScriptTM III first-strand synthesis supermix kit. Gene expression of ACAN (F: 5′-GCCTGCGCTCCAATGACT-3′, R: 5′-TAATGGAACACGATGCCTTTCA-3′, NM_001135), COL2A1 (F: 5′-GGCAATAGCAGGTTCACGTACA-3′, R: 5′-CGATAACAGTCTTGCCCCACTT-3′, NM_001844), COL1A1 (F: 5′-CAGCCGCTTCACCTACAGC-3′, R: 5′-TTTTGTATTCAATCACTGTCTTGCC-3′, NM_000088) and COL10A1 (F: 5′-ACCCAACACCAAGACACAGTTCT-3′, R: 5′-TCTTACTGCTATACCTTTACTCTTTATGGTGTA-3′, NM_000493) were analysed with real-time PCR using the SYBR GreenERTM qPCR supermix universal kit. All reagents and kits were purchased from Life Technologies, and samples were processed according to the manufacturer’s instructions. The cycle threshold ( C t ) value of each gene was normalized to the housekeeping gene β2 microglobulin (B2M, F: 5′-ATGAGTATGCCTGCCGTGTGA-3′, R: 5′-GGCATCTTCAAACCTCCATGATG-3′) using the comparative C t method (2 −Δ C t ). Glycosaminoglycan analysis Samples from the compression experiment were digested in 0.5 mg ml −1 proteinase K solution overnight at 60 °C ( n =5). Digested samples were analysed for GAG using the 1, 9-dimethylmethylene blue assay at pH 3. GAG measurements for each construct were normalized to its wet weight. Immunohistochemistry After 28 days, the reinforced GelMA-HA gels were paraffin-embedded and sectioned at 5 μm. For antigen retrieval, ready-to-use proteinase K solution (Dako) was used for 10 min at 37 °C. Sections were blocked with 2% FBS solution before exposure to primary antibodies: I-8H5 (MP Biomedicals), dilution 1:300 for collagen type I; II-II6B3 (DSHB), dilution 1:200 for collagen type II. Following incubation in fluorescence-labelled goat anti-mouse secondary antibody (Alexa Fluor 488, Invitrogen), sections were mounted with Prolong Gold (Invitrogen) and visualized using a confocal fluorescence microscope (A1R Confocal, Nikon). Statistics All data were expressed as mean±s.d. of five independent samples, unless stated otherwise. One-way analysis of variance (ANOVA) with Bonferroni correction was performed to compare the stiffness of the reinforced hydrogels; the effect of scaffold porosity was compared for every hydrogel and the effect of the hydrogel was compared for every scaffold porosity. Two-way ANOVA was used to evaluate the effect of compression and hydrogel types on gene expression, GAG/ww and stiffness. An independent samples t- test, not assuming equal variances, was performed to evaluate cell viability (SPSS, IBM software, USA). Differences were considered significant when P <0.05. How to cite this article : Visser, J. et al. Reinforcement of hydrogels using three-dimensionally printed microfibres. Nat. Commun. 6:6933 doi: 10.1038/ncomms7933 (2015).